Kondo physics in non-local metallic spin transport devices The non-local spin-valve is pivotal in spintronics, enabling separation of charge and spin currents, disruptive potential applications and the study of pressing problems in the physics of spin injection and relaxation. Primary among these problems is the perplexing non-monotonicity in the temperature-dependent spin accumulation in non-local ferromagnetic/non-magnetic metal structures, where the spin signal decreases at low temperatures. Here we show that this effect is strongly correlated with the ability of the ferromagnetic to form dilute local magnetic moments in the NM. This we achieve by studying a significantly expanded range of ferromagnetic/non-magnetic combinations. We argue that local moments, formed by ferromagnetic/non-magnetic interdiffusion, suppress the injected spin polarization and diffusion length via a manifestation of the Kondo effect, thus explaining all observations. We further show that this suppression can be completely quenched, even at interfaces that are highly susceptible to the effect, by insertion of a thin non-moment-supporting interlayer. Spintronic devices based on metals and insulators have been remarkably successful, as illustrated by the universal use of spin-valves, and now magnetic tunnel junctions, in hard disk read sensors. The need to scale such devices to extremely small sizes introduces serious impedance matching and noise issues, however, making all-metallic structures (for example, current-perpendicular-to-plane giant magnetoresistance stacks) [1] attractive for next-generation devices [2] . Remarkably, despite the maturity of metallic spintronics, there remain large gaps in our fundamental understanding of spin transport in metals, particularly with injection of spins across ferromagnet (FM)/non-magnetic metal (NM) interfaces, and their subsequent diffusion and relaxation. Unresolved issues include the applicability of the widely employed Elliott-Yafet (E-Y) [3] spin relaxation mechanism [4] , [5] , [6] , [7] , [8] , [9] , [10] , the influence of defects, surfaces and interfaces on spin relaxation at nanoscopic dimensions [8] , [11] , [12] , [13] , [14] , [15] , the importance of magnetic and spin-orbit scattering [16] , [17] , [18] and the accuracy of existing models [19] , [20] , [21] , [22] , [23] . In the quest to understand such issues, the non-local spin valve (NLSV) [24] has a pivotal role as it enables separation of charge and spin currents, providing a direct means to study spin injection, transport and relaxation [25] . In the NLSV geometry, two nanoscopic FM electrodes separated a distance d are electrically connected via a nanoscopic NM (that is, para- or dia-magnetic) channel. A spin-polarized charge current I Q is injected from one FM (FM inj ), and extracted from the far edge of the NM, away from the second FM electrode (FM det ). Ideally, in this geometry, no charge current flows between the two FM contacts. A non-equilibrium spin polarization thus accumulates above FM inj and diffuses, in both directions, along the NM channel, generating a diffusive pure spin current ( I S ) between FM inj and FM det . Some fraction of the injected spins reach FM det , generating a non-local spin-dependent potential difference, V NL (and a non-local resistance, R NL =V NL /I Q ) between FM det and the right edge of the NM. The magnetizations of FM inj and FM det are then switched between parallel (P) and antiparallel (AP) to determine ΔR NL =R P – R AP , a direct measure of the spin accumulation at FM det , devoid of complications due to charge currents. ΔR NL (d) can then be used to determine, via an appropriate model [19] , [21] , [22] , [25] , parameters such as the spin polarization of the injected current ( α ) and the NM spin diffusion length ( λ N ). This non-local geometry has enabled significant advances in the understanding of spin transport in metals [4] , [5] , [6] , [7] , [8] , [9] , [10] , [11] , [12] , [13] , [14] , [15] , [16] , [18] , [22] , [24] , [25] , [26] , [27] , [28] , [29] , [30] , [31] , [32] , [33] , [34] , [35] , [36] , [37] , but has also highlighted serious discrepancies with theory. The primary example of the latter is the surprising non-monotonicity in the temperature ( T ) dependence of ΔR NL , and thus the deduced λ N , in the transparent interface limit. In the widely investigated Ni 80 Fe 20 /Cu, for example, ΔR NL initially increases on cooling but then drops (by 10–40%, dependent on dimensions) below ~40 K (refs 8 , 10 , 18 , 30 , 31 , 32 , 33 ). This is in stark contrast to expectations from the E-Y mechanism [17] , [38] , which posits τ s ∝ τ p (where τ s is the NM spin lifetime and τ p the momentum relaxation time), that is, that spin relaxation occurs with finite probability at each momentum scattering event (~1 × 10 −3 for pure Cu [38] ). A monotonic decrease in NM resistivity ( ρ N ) on cooling implies a monotonic increase in τ p , and thus a monotonic increase in τ s and λ N , in direct contradiction with observations. This anomalous behaviour has proven very difficult to explain. Surface spin relaxation [10] , reduced dimensions [9] and surface [18] /bulk [8] (magnetic) impurities have all been advanced, but no consensus has emerged. One issue contributing to this is the focus on only a small set of materials, with Ni 80 Fe 20 /Cu and Ni 80 Fe 20 /Ag accounting for a major fraction of prior work [10] , [18] , [28] , [30] , [31] , [32] , [33] , [34] , [35] , [39] . In this work, via systematic studies significantly expanding the range of FM and NM materials investigated (encompassing Ni 80 Fe 20 , Ni, Fe, Co, Cu and Al), we show that in devices where the FM and NM are synthesized in a single deposition sequence, the low T downturn in ΔR NL is not a property of an individual NM but rather of the FM/NM pair. NM materials that do not support local magnetic moments when a given FM is diluted in them are found to show no low T anomalies, exemplified by Al. For the FM/NM pairs that do exhibit the anomalous non-monotonicity, we provide strong evidence that FM/NM interdiffusion leads to the formation of local moments which suppress α , and to a lesser extent λ N , via a manifestation of the Kondo effect. We further show that this suppression can be quenched by ultra-thin non-moment-supporting interlayers (ILs). We argue that these concepts provide a coherent explanation of all major features of the available data, with implications even for room temperature spin transport. Field dependence of the non-local resistance A schematic of the NLSV geometry employed in our work is shown in Fig. 1a ; a typical ( d= 250 nm) NLSV device is shown in the scanning electron microscope image of Fig. 1b . The FM electrodes have widths w FM,inj and w FM,det , and thickness t FM , whereas the NM channel has width w N and thickness t N . Unless otherwise noted, devices in this work have t FM =16 nm and t N =200 nm. In Fig. 1c,d , we first illustrate the basic response of R NL to in-plane and perpendicular-to-plane magnetic fields ( H || and H ⊥ , Fig. 1a ). 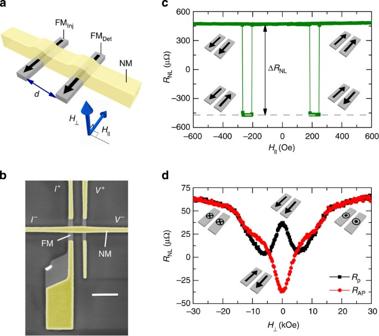Figure 1: Non-local spin valve experimental geometry and field-dependence of the non-local resistanceRNL. (a) Schematic of the experimental NLSV geometry showing ferromagnet (FM) and non-magnetic metal (NM) materials, the inter-FM separation (d) and the field orientation for parallel,H||,and perpendicular,H⊥,alignment. (b) False colour scanning electron microscope image of ad=250 nm Fe/Cu device showing current (I) and voltage (V) contact orientations (with a 500 nm scale bar). (c) In-plane field dependence ofRNLfor a Ni80Fe20/Al device withd=250 nm at temperature,T=50 K, with ΔRNL=RP−RAPindicated. (d) Out-of-plane (Hanle geometry) field dependence of the parallel,RP(black squares), and anti-parallel,RAP(red circles), non-local resistance for an Fe/Cu device withd=2 μm atT=50 K. The schematic labels shown in (c,d) indicate the orientation of FM injector and detector. Figure 1c shows R NL ( H || ) for a d= 250 nm Ni 80 Fe 20 /Al device at T= 50 K, the labels showing the magnetization orientation of FM inj and FM det . As is typical [26] , a small field-independent background (16 μΩ here) has been subtracted. Complete and abrupt switching between P and AP is observed, enabling determination of ΔR NL , the T and d dependence of which allow for extraction of α ( T ) and λ N ( T ). Figure 1d shows the dependence of R P and R AP on H ⊥ , for a d= 2 μm Fe/Cu device at T= 50 K. The gradually damped oscillations derive from the Hanle effect [12] , [23] , [25] , [29] , [36] , [37] , [39] (because of the precession of the diffusing spins about H ⊥ ), R P and R AP merging at high H ⊥ when FM inj and FM det are driven out of plane (see schematics, Fig. 1d ). Such data enable extraction of τ s , and thus (where D is the electron diffusivity), complementary to that from ΔR NL ( d ). Figure 1: Non-local spin valve experimental geometry and field-dependence of the non-local resistance R NL . ( a ) Schematic of the experimental NLSV geometry showing ferromagnet (FM) and non-magnetic metal (NM) materials, the inter-FM separation ( d ) and the field orientation for parallel, H ||, and perpendicular, H ⊥ , alignment. ( b ) False colour scanning electron microscope image of a d= 250 nm Fe/Cu device showing current ( I ) and voltage ( V ) contact orientations (with a 500 nm scale bar). ( c ) In-plane field dependence of R NL for a Ni 80 Fe 20 /Al device with d= 250 nm at temperature, T= 50 K, with ΔR NL =R P −R AP indicated. ( d ) Out-of-plane (Hanle geometry) field dependence of the parallel, R P (black squares), and anti-parallel, R AP (red circles), non-local resistance for an Fe/Cu device with d= 2 μm at T= 50 K. The schematic labels shown in ( c , d ) indicate the orientation of FM injector and detector. Full size image Varying FM/NM material combinations Before detailed analysis of α ( T ), λ N ( T ) and τ s ( T ), we first present a central observation of this work, arrived at by studying ΔR NL ( T ) in a large set of materials ( Fig. 2 ). The data are from NLSVs with d= 250 nm, and a logarithmic T axis is chosen to illustrate the low T behaviour. 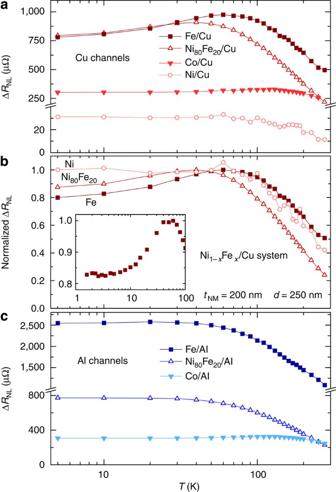Figure 2: Temperature dependence of the spin accumulation signal for various ferromagnet/non-magnetic metal material pairings. (a) Spin accumulation signal, ΔRNL, as a function of temperature,T,(log scale) for various ferromagnet FM materials, using Cu (red data) as the non-magnetic metal NM channel material. The FM contact material is indicated by: Fe, closed squares; Ni80Fe20, open triangles; Co, closed triangles; Ni, open circles. (b) Normalized ΔRNLas a function ofTfor the Ni1−xFex/Cu system. The inset shows a plot of the normalized ΔRNLversusTat low temperatures for Fe/Cu, highlighting the saturation asT→0. (c) ΔRNL, as a function ofT(log scale) for various FM materials, using Al (blue data) as the NM channel material. All displayed data are obtained fromd=250 nm devices, with NM thickness,tNM=200 nm. Figure 2a focuses on Cu channels with Fe, Ni 80 Fe 20 , Co and Ni, Fig. 2b on Cu channels with Ni 100- x Fe x ( x= 0, 20 and 100), and Fig. 2c on Al with Fe, Ni 80 Fe 20 and Co. Beginning with Fig. 2a , we first note the ΔR NL ( T ) for Ni 80 Fe 20 /Cu, which indeed shows the anomalous decrease below ~40 K (refs 8 , 10 , 18 , 30 , 31 , 32 , 33 ). Considering Co, Fe and Ni, however, it can be seen that the low T downturn in ΔR NL ( T ) is obviously not a property of the NM alone, but is strongly influenced by the FM. Specifically, Fe/Cu shows the strongest downturn (onset temperature of 60 K), followed by Ni 80 Fe 20 /Cu (40 K onset), and then Co/Cu, where the effect is weak but occurs below ~130 K. In Ni/Cu on the other hand, we find no evidence for a low T downturn in ΔR NL ( T ). The Ni 100− x Fe x /Cu case is particularly interesting and is highlighted in Fig. 2b , where data for Ni, Ni 80 Fe 20 and Fe are shown normalized to the maximum ΔR NL . A clear progression is apparent. One interpretation, which we return to below, is that the low T downturn in ΔR NL ( T ) only occurs in Ni 80 Fe 20 /Cu because of the presence of Fe. Additional important information is obtained by extending the T range down to ~1 K. As shown in the inset to Fig. 2b (for Fe/Cu), the suppression of ΔR NL in fact saturates at low T , below ~5 K in this case. Finally, turning to Fig. 2c , we find radically different behaviour with Al channels. In Al devices, no significant low T suppression is observed for any FM, ΔR NL ( T ) monotonically increasing on cooling, qualitatively consistent with the E-Y mechanism. A number of other trends are also apparent in Fig. 2 , such as the influence of the FM on the high T behaviour. The T dependence in this region strengthens as the FM is varied from Ni 80 Fe 20 →Ni→Fe→Co, which we ascribe to the influence of Curie temperature ( T C ) and magneto-crystalline anisotropy on α ( T ). FMs such as Co, with high T C and relatively large anisotropy, are expected to present weak α ( T ), whereas FMs such as Ni 80 Fe 20 and Ni, with lower T C and anisotropy, should have stronger α ( T ) [40] . A second observation is the large variation in ΔR NL ( T= 0), which spans 30–2,500 μΩ. Although a number of factors contribute, particularly the resistivities of the FM and NM ( ρ FM and ρ N ), α ( T= 0) is a dominant parameter. It accounts in particular for the low ΔR NL in Ni, where α is significantly smaller than in Co, Ni 80 Fe 20 and Fe (refs 41 , 42 ). Figure 2: Temperature dependence of the spin accumulation signal for various ferromagnet/non-magnetic metal material pairings. ( a ) Spin accumulation signal, ΔR NL , as a function of temperature, T, (log scale) for various ferromagnet FM materials, using Cu (red data) as the non-magnetic metal NM channel material. The FM contact material is indicated by: Fe, closed squares; Ni 80 Fe 20 , open triangles; Co, closed triangles; Ni, open circles. ( b ) Normalized ΔR NL as a function of T for the Ni 1−x Fe x /Cu system. The inset shows a plot of the normalized ΔR NL versus T at low temperatures for Fe/Cu, highlighting the saturation as T →0. ( c ) ΔR NL , as a function of T (log scale) for various FM materials, using Al (blue data) as the NM channel material. All displayed data are obtained from d= 250 nm devices, with NM thickness, t NM =200 nm. Full size image Fitting ΔR NL (d) and the Hanle effect To further investigate such issues, particularly the low T decrease in ΔR NL , α ( T ) and λ N ( T ) were extracted from ΔR NL ( d , T ), focusing on Fe/Cu (with the strongest downturn) and Fe/Al (no downturn). Such data are shown in Fig. 3a,b , where ΔR NL ( d ) is plotted at various T . 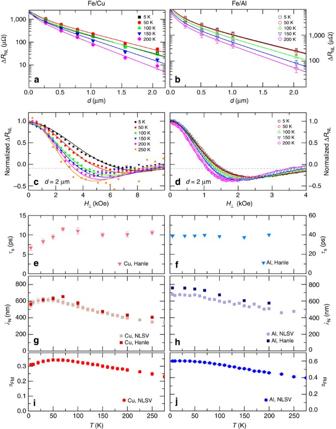Figure 3: Comparison between fitted parameters from Hanle and non-local spin valve (NLSV) geometries for Fe/Cu (left column, closed symbols) and Fe/Al (right column, open symbols) devices. (a,b) Ferromagnet (FM) separation (d) dependence of spin accumulation signal, ΔRNL,for various temperatures,T. Solid lines are fits using the 1-D Valet-Fert model described in the text, constraining the ferromagnet spin diffusion length,λFM, to 4 nm. Error bars are the estimated total uncertainty obtained by combining in quadrature the standard error in the spin accumulation signal with systematic uncertainties in the device geometry. (c,d) Perpendicular magnetic field,H⊥, dependence of ΔRNL(Hanle geometry), normalized to ΔRNL(H⊥=0), for variousT. Solid lines are fits using a 1-D spin diffusion model including: effects of finite contact width, rotation of FMs and diffusivity,D(T),determined from the non-magnetic metal (NM) resistivity,ρN(T). The grey dashed line indicates ΔRNL=0. (e,f) NM spin lifetime,τs, obtained from fitting Hanle effect data (c,d). (g,h) Comparison of NM spin diffusion length,λN(T),obtained from fitting the NLSV separation dependence (lighter colors;λFM=4 nm) and Hanle effect measurements (darker colours;D(T)constrained byρN(T)). (i,j) Current polarization,α, obtained from fitting NLSV separation dependence. The solid lines are fits using an analytical solution [20] , [21] to the NLSV spin diffusion problem in 1-D: Figure 3: Comparison between fitted parameters from Hanle and non-local spin valve (NLSV) geometries for Fe/Cu (left column, closed symbols) and Fe/Al (right column, open symbols) devices. ( a , b ) Ferromagnet (FM) separation ( d ) dependence of spin accumulation signal, ΔR NL, for various temperatures, T . Solid lines are fits using the 1-D Valet-Fert model described in the text, constraining the ferromagnet spin diffusion length, λ FM , to 4 nm. Error bars are the estimated total uncertainty obtained by combining in quadrature the standard error in the spin accumulation signal with systematic uncertainties in the device geometry. ( c , d ) Perpendicular magnetic field, H ⊥ , dependence of ΔR NL (Hanle geometry), normalized to ΔR NL (H ⊥ =0) , for various T . Solid lines are fits using a 1-D spin diffusion model including: effects of finite contact width, rotation of FMs and diffusivity, D(T), determined from the non-magnetic metal (NM) resistivity, ρ N (T) . The grey dashed line indicates ΔR NL =0 . ( e , f ) NM spin lifetime, τ s , obtained from fitting Hanle effect data ( c , d ). ( g , h ) Comparison of NM spin diffusion length, λ N (T), obtained from fitting the NLSV separation dependence (lighter colors; λ FM =4 nm) and Hanle effect measurements (darker colours; D(T) constrained by ρ N (T) ). ( i , j ) Current polarization, α , obtained from fitting NLSV separation dependence. Full size image where α = I ↑ − I ↓ / I ↑ + I ↓ is the current polarization of the FM, λ FM is the spin diffusion length in the FM, and R N =ρ N λ N /w N t N and R FM =ρ FM λ FM /w FM w N are the N and FM spin resistances. This expression applies in the transparent interface limit, that is, interface resistance < R N , R FM , which we verify to be the case here (see Supplementary Figs 1 and 2 and Supplementary Notes 1 and 2 ). All geometrical parameters in equation (1) were measured for each device, as were ρ N ( T ) and ρ FM ( T ) (see Supplementary Fig. 2 and Supplementary Note 2 ). This nevertheless leaves α ( T ), λ FM ( T ) and λ N ( T ) as free parameters, resulting in poorly constrained fitting. Specifically, although λ N ( T ) determines the d dependence of ΔR NL , and can be independently extracted (particularly in the d > λ N limit where an exponential fall-off is recovered), α ( T ) and λ FM ( T ) control the magnitude of ΔR NL and are inseparable, entering through λ FM /(1− α 2 ). Constraints on one of λ FM or α are thus required. As a starting point, we simply hold λ Fe constant at 4 nm, a value determined from the measured ρ Fe ( T= 5 K) via the observed scaling between λ FM and ρ FM [43] . The resulting λ N ( T ) is shown in Fig. 3g,h , labelled as ‘Cu, NLSV’ and ‘Al, NLSV’, while α ( T ) is shown in Fig. 3i,j . In the Fe/Al case, both α and λ N increase monotonically on cooling. However, Fe/Cu is more complex. As shown in Fig. 3g , λ N ( T ) increases down to 50 K, below which it appears to undergo a slight decrease. This decrease is barely above experimental uncertainty, however, amounting to 6±6% based on our best error estimates. In contrast, a clear and statistically significant decrease in α is found as T is lowered below 50 K ( Fig. 3i ). As ΔR NL at d= 250 nm is more sensitive to α than λ N (from equation (1), see Supplementary Fig. 3 and Supplementary Note 3 ), this 15% decrease in α corresponds to a 28% decrease in ΔR NL , the majority of the observed suppression. We thus conclude that the low T downturn in ΔR NL in our NLSVs, although containing some contribution from enhanced spin relaxation, is dominated by d -independent suppression of the spin injection/detection efficiency. Exhaustive fitting, with a multitude of parameter constraints (see Supplementary Fig. 3 and Supplementary Note 3 ), confirms this. As discussed above, R NL ( H ⊥ ), via the Hanle effect, provides access to τ s , and an independent check of λ N ( T ). In Fig. 3c,d , we thus plot ΔR NL ( H ⊥ )=[ R P ( H ⊥ )− R AP ( H ⊥ )]/[ R P (0)− R AP (0)], at various T , for Fe/Cu and Fe/Al at d= 2 μm. (This was recorded for positive and negative H ⊥ , but we plot here only the symmetric component.) Such large d is used to enable fitting with analytical expressions for spin diffusion-precession (see Methods), with no need to account for back-diffusion of injected spins [23] . The width and amplitude of the oscillations in Fig. 3c,d are controlled solely by τ s and D , and the fits (solid lines) use D ( T ) determined from the measured ρ N ( T ), resulting in the τ s ( T ) shown in Fig. 3e,f . For both Fe/Cu and Fe/Al, τ s is remarkably flat above 70 K, a dramatic illustration of the dominance of defects (for example, non-magnetic point-defects, grain boundaries) in spin relaxation. In accord with the E-Y mechanism, T -independent momentum relaxation processes associated with such defects result in T -independent spin relaxation. For Fe/Cu only ( Fig. 3e ), the situation is markedly different below 70 K, where τ s drops from 12 to 7 ps, clearly correlated with ΔR NL ( T ). Despite this substantial decrease in τ s , the corresponding drop in ( Fig. 3g , ‘Cu, Hanle’) is small due to the increase in D (from 1/ ρ N ) on cooling. The overall agreement between λ N determined from ΔR NL ( d ) and from the Hanle effect is excellent ( Fig. 3g,h ), and the form of λ N ( T ) for Fe/Cu is confirmed. The observation that the downturn in ΔR NL ( T ) in our devices is dominated by α ( T ) (with only a secondary contribution from λ N ( T )), and is highly sensitive to the FM/NM pairing, is inconsistent with ‘channel only’ explanations, such as surface spin relaxation. This is underscored by the additional observation (for example, in Ni 80 Fe 20 /Cu, Supplementary Fig. 4 and Supplementary Note 4 ) that the ΔR NL suppression is t N independent [8] . Rather, the dominance of α ( T ) and sensitivity to FM/NM pairing point to explanations based on low T suppression of spin injection/detection efficiency at the interfaces. One general possibility for such is the formation of non-trivial interfacial magnetic states at low T because of FM/NM interdiffusion, such as spin-glass-like interfaces (potentially depolarizing the injected spin current), or non-collinear states (preventing full polarization). To investigate such possibilities, we undertook detailed T -dependent polarized neutron and X-ray reflectivity measurements on Ni 80 Fe 20 /Cu and Co/Cu bilayers deposited under identical conditions to our NLSVs. The data ( Supplementary Figs 5 and 6 and Supplementary Notes 5 and 6 ) reveal remarkably T -independent magnetic depth profiles, however, ruling out even minor changes in the interfacial magnetic structure at low T . In Ni 80 Fe 20 /Cu, for example, the magnetic interface width is only 0.6 nm, with no apparent T dependence. Local moments and the Kondo effect in spin transport This confinement of strong FM/NM intermixing to a thin region close to the interface does not, however, rule out explanations based on low densities of FM impurities in the NM, whether from interdiffusion, residual FM vapour pressure during NM deposition, contamination of the NM source material [8] or other sources [18] . Table 1 , which compares the ability of Cu and Al to host local magnetic moments when the FMs used in this work are added as dilute impurities, reveals some striking correlations in this context. 3 d elements form local moments only when diluted in certain NMs [44] , [45] , [46] , a fact that can be understood within the Anderson virtual bound state model [44] , [45] , where the local moment is dictated by the relative magnitudes of the NM Fermi energy ( E F ), s - d hybridization potential and FM intra-atomic d-d Coulomb repulsion. In Al, for example, the high E F locates both up-spin and down-spin virtual bound states below the Fermi surface, quenching local moments [44] , [45] , [46] . Considering Table 1 , the correlation between local moment formation and the occurrence of a low T downturn in ΔR NL ( T ) in a given FM/NM pair is in fact striking, the only apparent anomaly being Ni/Cu, as discussed below. Table 1 Comparison between the Kondo temperature T K and the T at which a maximum in Δ R NL (T) occurs, T max . Full size table Importantly, in the cases where local moments do form, the Kondo effect [44] , [45] , [46] , [47] , [48] , [49] is anticipated. Essentially, delocalized electrons in the NM are expected to screen the local moments from dilute FM impurities around some characteristic T scale, T K (refs 45 , 46 ). Table 1 shows not only that the downturn in ΔR NL ( T ) correlates with the formation of local moments, but moreover, that the observed downturn temperature ( T max ) correlates with T K . For Ni in Cu, for example, although dilute moments form, the extremely high T K (>1,000 K) precludes observation of Kondo physics at T ≤300 K, consistent with observations. For Fe in Cu on the other hand, T K =30 K (ref. 44 ), comparing reasonably to T max =60 K for Fe/Cu and T max =40 K for Ni 80 Fe 20 /Cu. Note that in the latter case, because of the prohibitively high T K for Ni in Cu, only Fe impurities contribute to the changes of ΔR NL (T) over the measured T range, consistent with the larger downturn in Fe than Ni 80 Fe 20 ( Fig. 2b ). For Co in Cu, we observe only a weak downturn, with T max =130 K. The limited solubility in this case limits the strength of Kondo effects, whereas the 130 K T max is consistent with the 23 K< T K <500 K bound from known limits for surface and bulk Co impurities in Cu (refs 44 , 47 ). This Kondo-suppressed spin accumulation picture is also consistent with literature observations in the heavily studied Ni 80 Fe 20 /Ag system [5] , [29] , [35] , [36] , including the existence of a downturn (because of local Fe moments in Ag), the relatively weak decrease in ΔR NL (7%, because of low miscibility) and the approximate correspondence between T max (<20 K) and T K (~5 K for Fe/Ag). Taken as a whole, the correlations between moment formation, T K , and the magnitude and onset temperature of the downturn in ΔR NL are thus remarkably strong across a wide variety of materials, revealing a simple pattern to the apparently complexity in Fig. 2 . Given these strong correlations with moment formation, miscibility and T K , we propose a scenario where dilute quantities of FM impurities in the near-interface region of the NM lead to a novel manifestation of the Kondo effect. We suggest that the disordered local moments (and the accompanying conduction electron screening) depolarize the injected spin current at temperatures around T K , reducing the polarization injected into the bulk of the channel (see Supplementary Fig. 7 and Supplementary Note 7 ). Although such physics has not been previously discussed in NLSVs, the reciprocal role of spin injection on the Kondo effect in charge transport has been explored [48] , and some precedent for related effects exists in magnetic tunnel junctions [50] . Critically, we believe that this picture provides qualitative explanations for all observed phenomena. The absence of a downturn in Al-based devices, the miscibility-related magnitude in FM/Cu and the correlation between T max and T K are all straightforwardly understood. Regarding the latter it should be noted that in this picture T max will be determined by the competition between the Kondo suppression of the spin accumulation and the usual α ( T ), λ ( T ) and ρ ( T ), meaning that the correlation between T K and T max is expected to be only approximate, as is the case. Our model also explains the saturation of the downturn in ΔR NL ( T ) at very low T in Fe/Cu ( Fig. 2b , inset), as the Kondo suppression of α should saturate at T << T K , because of inter-moment d–d interactions and entry into the unitary scattering limit [44] , [45] , [46] . Note that the fact that we observe no conventional Kondo effect in direct four-terminal ρ N ( T ) measurements on our devices (see Supplementary Figs 2 and 4 and Supplementary Notes 2 and 4 ) in no way contradicts this picture. The charge current in such measurements will be dominated by the highest conductivity central regions of the NM channel, the near-interface regions relatively rich in FM impurities having little influence on ρ N ( T ). This would be expected to change if interdiffusion were promoted to the extent that the bulk of the NM channel reached FM concentrations > O (1 p.p.m. ), where the Kondo effect emerges. To demonstrate this directly, we thermally annealed a d= 250 nm Fe/Cu device for 2 h under high vacuum at 500 °C, resulting in the ρ N ( T ) shown in the inset of Fig. 4a , where a clear Kondo minimum occurs. The ρ N ( T ) curve can in fact be fit to an empirical relation [51] for the Kondo effect (purple solid line, see Methods) with T K =30 K, yielding a Kondo resistivity, ρ K =0.06 μΩcm, and a resistivity minimum at 20.5 K. The latter is consistent with an average Fe concentration of 100–200 p.p.m. (ref. 52 ). Most importantly, examining ΔR NL ( T ) for such a device ( Fig. 4a ), we find a substantial enhancement of the downturn, ΔR NL being reduced by ~50% below a T max that now exceeds 100 K. These results prove that Kondo physics is active in charge transport in our devices and that the anomaly in ΔR NL ( T ) is indeed enhanced as the charge Kondo effect is promoted, as expected. 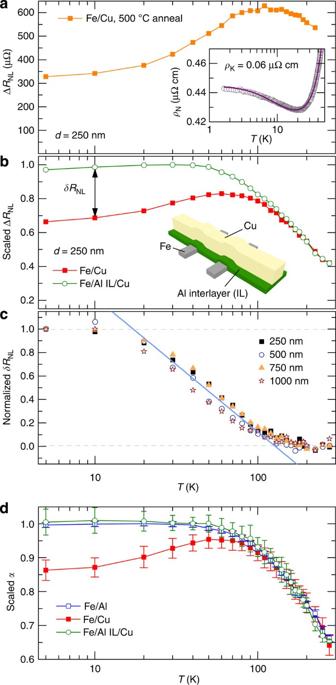Figure 4: Effect of annealing and Al interlayer insertion on spin transport. (a) Spin accumulation signal, ΔRNL, as a function of temperature,T, for an Fe/Cu device with ferromagnet separation,d=250 nm, annealed at 500 °C under high vacuum for 2 h. Inset: an example of non-magnetic metal (NM) resistivity,ρN(T), for such a device (grey circles), demonstrating a Kondo upturn. Data are fit using an empirical Kondo model (purple solid line). (b)Tdependence of ΔRNLford=250 nm Fe/Cu devices (solid red squares) and devices with an ~5-nm thick Al interlayer (Fe/Al IL/Cu, green open circles). Values are scaled to Fe/Al IL/Cu at high-T(T>150 K) for comparison. Inset: schematic of the non-local spin valve geometry with a thin (~5 nm) Al interlayer between the FM and NM. (c) Difference in ΔRNLbetween Fe/Cu and Fe/Al IL/Cu devices,δRNLas a function ofT, for various FM separations,d. Solid line is a fit of all data toδRNL=a[1–b log(T/TK)], whereTKis the Kondo temperature for Fe/Cu anda, bare free parameters. (d) Comparison of current polarization,α(T),obtained from fitting the NLSV separation dependence for Fe/Al (open blue squares), Fe/Cu (solid red squares) and Fe/Al IL/Cu (open green circles). All values are scaled to the Fe/Al high-Tdata for comparison. Error bars on the fit parameters are the standard errors from a least squares fit of the experimental data (appropriately weighted by combining in quadrature the standard error in the spin accumulation signal with systematic uncertainties in the device geometry). Figure 4: Effect of annealing and Al interlayer insertion on spin transport. ( a ) Spin accumulation signal, ΔR NL , as a function of temperature, T , for an Fe/Cu device with ferromagnet separation, d= 250 nm, annealed at 500 °C under high vacuum for 2 h. Inset: an example of non-magnetic metal (NM) resistivity, ρ N ( T ), for such a device (grey circles), demonstrating a Kondo upturn. Data are fit using an empirical Kondo model (purple solid line). ( b ) T dependence of ΔR NL for d= 250 nm Fe/Cu devices (solid red squares) and devices with an ~5-nm thick Al interlayer (Fe/Al IL/Cu, green open circles). Values are scaled to Fe/Al IL/Cu at high- T ( T >150 K) for comparison. Inset: schematic of the non-local spin valve geometry with a thin (~5 nm) Al interlayer between the FM and NM. ( c ) Difference in ΔR NL between Fe/Cu and Fe/Al IL/Cu devices, δR NL as a function of T , for various FM separations, d . Solid line is a fit of all data to δR NL =a[1–b log(T / T K )], where T K is the Kondo temperature for Fe/Cu and a, b are free parameters. ( d ) Comparison of current polarization, α(T), obtained from fitting the NLSV separation dependence for Fe/Al (open blue squares), Fe/Cu (solid red squares) and Fe/Al IL/Cu (open green circles). All values are scaled to the Fe/Al high- T data for comparison. Error bars on the fit parameters are the standard errors from a least squares fit of the experimental data (appropriately weighted by combining in quadrature the standard error in the spin accumulation signal with systematic uncertainties in the device geometry). Full size image A final point to emphasize regarding the Kondo suppression of ΔR NL ( T ) is that while in our case the role of α ( T ) is dominant over λ N ( T ), this balance could vary with synthesis conditions. Deposition of the FM and NM in separate systems [10] , contamination of the NM source with FM impurities [53] and transfer of FM impurities to the NM channel from resists [18] will change the balance between FM/NM interface and bulk channel magnetic impurity contributions, altering the relative contributions of α ( T ) and λ N ( T ) to the downturn in ΔR NL . Quenching local moments and restoring ΔR NL (T) Having identified the Kondo effect at FM/NM interfaces as the key factor in the low T downturn in ΔR NL , it is natural to consider whether this effect, which is deleterious in terms of maximizing spin signals, can be mitigated. Although it is clear that pure Al channels provide one means to do so, a more general approach, compatible with any channel material, would be preferable. To this end, we pursued insertion of thin Al ILs between FM and NM, the low solubility of transition metal FMs in Al minimizing interdiffusion, whereas the properties of Al eliminate local moment formation and Kondo effects. Fe/Cu NLSVs were thus fabricated with a ~5-nm thick IL between the Fe and Cu (see Methods, and the schematic in Fig. 4b ). Simple calculations establish that contributions to the spin transport from the IL in comparison to the bulk of the Cu channel can safely be neglected ( Supplementary Fig. 8 and Supplementary Note 8 ). Figure 4b compares ΔR NL at d= 250 nm for Fe/Cu and Fe/Al IL/Cu devices. The data are scaled to overlap at high T (>150 K), in order to easily assess the impact of the Al IL on the low T ΔR NL . Remarkably, the low T Kondo suppression of the spin accumulation is almost completely removed by an IL of only 5 nm. Defining δR NL as the difference between the high- T -scaled ΔR NL ( T ) for Fe/Al IL/Cu and Fe/Cu devices ( Fig. 4b ), we plot in Fig. 4c δR NL ( T ), normalized to its 5 K value, for several d . Not only do the data collapse to a single universal curve, but also, as demonstrated by the fit, the behaviour around T K is well described by logarithmic scaling. Specifically, the solid line is a fit to δR NL =a [1– b log ( T / T K )] with T K =30 K, the accepted value for Fe in Cu. Such a logarithmic form around T K , with expected negative and positive deviations below and above T K , respectively, is a commonly used phenomenological description of Kondo physics [44] , [50] , and can be rationalized from equation (1) assuming δα ∝ [ 1 – A log ( T / T K )], that is, a Kondo-related suppression of α . An understanding beyond simple phenomenology will require an approach sophisticated enough to capture the T -dependent influence of local moments and their associated conduction electron screening, as was achieved in the normal Kondo effect via higher-order perturbation theory. That the effect we see here is certainly dominated by α, however, is emphasized in Fig. 4d , where α ( T ), scaled to its maximum value, is plotted for Fe/Al, Fe/Cu and Fe/Al IL/Cu. These data result from a large set of ΔR NL ( T , d ) data ( Supplementary Fig. 8 and Supplementary Note 8 ). The 5-nm thick IL in the Fe/Al IL/Cu device almost completely restores α ( T ) to the monotonic form found in Fe/Al. We note that tunnel barriers between the FM and NM [5] , [13] , [14] , [25] , [36] , [50] could have a similar role, provided they prevent even minor NM/FM contamination. In summary, we have proposed a solution to the long-standing puzzle of the non-monotonicity of the T -dependence of the spin accumulation signal in metallic NLSV devices, the essential concept being a novel manifestation of the Kondo effect. In essence, we propose that in FM/NM combinations where the FM forms local moments when diluted in the NM, Kondo screening of the spin-disordered local moments leads to suppression of the injection/detection efficiency, and to some extent the NM spin diffusion length, around the Kondo temperature. We have further demonstrated a simple means to mitigate this effect, via insertion of a thin non-moment-supporting layer between the FM and NM. In addition to providing a solution to this immediate problem, and posing a significant challenge for future theoretical work, we propose that this work also highlights a number of potential new directions at the interface between spintronics and Kondo physics [54] , [55] . We imagine future research to more fully explore the impact of Kondo physics on spin transport in metallic hetero- and nano-structures, as well as the reciprocal effects of spin injection and relaxation on Kondo systems. Significantly, the potential relevance of these ideas to room temperature spin transport should also be explored. Common systems such as Ni/Cu, Co/Cu and Co/Au possess very high Kondo temperatures, raising the possibility that physics of the type elucidated here could be suppressing spin accumulation even at room temperature. Device fabrication NLSV devices were fabricated on Si/Si-N(2,000 Å) substrates using a Vistec EBPG5000+ electron beam lithography tool with a PMGI/PMMA bilayer resist stack. Clean, transparent FM/NM interfaces were achieved by multi-angle deposition [7] , [37] , without breaking vacuum, with the FM deposited at an angle of 49° and the NM at normal incidence. That the transparent interface limit [20] , [21] , [22] was achieved was explicitly verified by FM/NM contact resistance, Hanle effect and ΔR NL ( d ) measurements (see Supplementary Figs 1 and 2 ). All materials were deposited in the same vacuum system (base pressure O (10 −10 Torr)), using electron beam (for Al, Co, Cu, Fe, Ni, Ni 80 Fe 20 ) or thermal (for Cu) evaporation. Deposition rates for NM and FM materials were 1.0 and 0.5 Å s −1 , respectively, with growth pressures from 8 × 10 −10 to 1 × 10 −8 Torr. Nominal purities for the FM and NM materials were 99.95% and 99.999%, respectively. Film thicknesses were calibrated using ex situ grazing incidence X-ray reflectivity and monitored during deposition using a quartz crystal monitor. Patterned wire widths and separations were directly measured via scanning electron microscopy ( w N =150–200 nm, w FM,inj =150 nm and w FM,det =100 nm). A domain wall nucleation pad was incorporated into FM inj to reduce its coercivity and enable the AP state to be reliably obtained. Transport measurements and fitting Transport measurements were performed with 13 Hz AC excitation, at bias currents from 100 μA to 1 mA. At low T , careful checks for self-heating were carried out. Measured ΔR NL values were corrected for small (<10%) sample-to-sample variations in ρ and w N using the scaling expected from equation 1. For Hanle measurements, data were acquired in both the P and AP states (as shown in Fig. 1d ). The difference between these two signals ( Fig. 3c,d ) removes any background associated with FM rotation and leaves only the spin precession component [37] . Note that the data presented in Fig. 3c,d are averages from positive and negative H ⊥ sweeps. These data were fit to a solution of the spin-precession-diffusion equation, taking into account finite contact size and rotation of the magnetization of the FM electrodes: where ω L is the Larmor frequency ( ω L =γB, with γ the gyromagnetic ratio and B the magnetic flux density), t is the spin transit time, S 0 is a scaling term to account for the zero-field spin signal and x det (x i nj ) accounts for integration of the signal over the finite detector (injector) contact width. Note that this model does not take into account the effect of back-diffusion of spins into the FMs (that is, spin sinking). However, by d -dependent Hanle measurements, we have verified that the large separations reported here ( d= 2 μm) are in the NM-channel-dominated regime, where spin sinking is negligible [23] . For fitting, D ( T ) is determined from the experimental ρ N ( T ) using a form of the Einstein relation, ρ N ( T ) − 1 =e 2 N ( E F ) D ( T ), where N ( E F ) is the density-of-states at the Fermi level. Note that the displayed curves ( Fig. 3c,d ) use a slightly suppressed M s to phenomenologically account for in-plane rotation and demagnetization of the FM electrodes. The fitting results are quite insensitive to this value of M s , however, and, although the fit quality suffers, using standard literature values for M s does give quantitatively similar results for τ s . The Fe/Cu devices for which data are shown in Fig. 4a were annealed in high vacuum (base pressure 10 −7 Torr). The low T resistivity was fit using a phenomenological model for the Kondo contribution to the resistivity [51] : with . ρ 0 describes the impurity scattering contribution to ρ , whereas A and B account for electron–electron and electron–phonon scattering. We fix s= 0.225 and T K =30 K from literature values to obtain the Kondo resistivity ρ K . IL device fabrication For the devices with an IL, a ~5-nm thick Al layer was grown after FM deposition. To ensure appropriate coverage of the FM/NM interface region (that is, a layer width> w N , see inset to Fig. 4a ), this was done in discrete steps between −3° and +3° from normal incidence. Al was chosen as the IL material for several reasons: Fe atoms that diffuse into Al will not form local moments; the diffusivity of Fe in Al is substantially lower than it is in Cu and the use of a thin ( t<<λ N ), low ρ N material such as Al should not otherwise alter the magnitude or T -dependence of the spin accumulation. How to cite this article: O’Brien, L. et al. Kondo physics in non-local metallic spin transport devices. Nat. Commun. 5:3927 doi: 10.1038/ncomms4927 (2014).